A stabilizing factor for mitochondrial respiratory supercomplex assembly regulates energy metabolism in muscle The mitochondrial respiratory chain is essential for oxidative phosphorylation and comprises multiple complexes, including cytochrome c oxidase, assembled in macromolecular supercomplexes. Little is known about factors that contribute to supercomplex organization. Here we identify COX7RP as a factor that promotes supercomplex assembly. Cox7rp -knockout mice exhibit decreased muscular activity and heat production failure in the cold due to reduced COX activity. In contrast, COX7RP -transgenic mice exhibit increased exercise performance with increased cytochrome c oxidase activity. Two-dimensional blue native electrophoresis reveals that COX7RP is a key molecule that promotes assembly of the III 2 /IV n supercomplex with complex I. Our study identified COX7RP as a protein that functions in I/III 2 /IV n supercomplex assembly and is required for full activity of mitochondrial respiration. The respiratory chain supercomplexes in the inner membrane of mitochondria form ‘respirasome’ structures, which mainly comprise complexes I and III, and the terminal enzyme COX (complex IV) in mammalian cells [1] , [2] . Complexes II and V are usually not associated with any of the other complexes [3] . Complex IV is comprised of three subunits encoded by mitochondrial DNA and 10 subunits encoded by nuclear DNA [4] . In addition to mutations in mitochondrial DNA-encoded COX genes [5] , [6] , mutations in nuclear DNA-encoded COX component genes and COX accessory factors cause COX deficiency [6] , [7] , [8] . For example, SURF1 is responsible for Leigh syndrome [9] , [10] , SCO1 for neonatal-onset hepatic failure and encephalopathy [11] , SCO2 for fatal infantile cardioencephalomyopathy [12] , and COX15 for fatal hypertrophic cardiomyopathy [13] . SCO1 and SCO2 are copper metallochaperones that are necessary for copper insertion into the catalytic core of COX assembly [14] . The latter has a particular role in the regulation of cellular copper homoeostasis as the overexpression of SCO2 can suppress cellular copper deficiency in fibroblasts from SCO2 , SCO1 and COX15 mutation patients [15] . Supercomplex assembly has been shown to enhance respiratory chain activity through spatial restriction of electron carrier diffusion [3] , although the factors involved in the formation and maintenance of supercomplex assembly remain to be elucidated. As a phospholipid that maintains the integrity of the mitochondrial membrane, cardiolipin is required for the specific association between complexes and a decrease in its content might deeply affect inter-complex assembly [16] . A mutation of the cardiolipin-remodeling enzyme TAZ forms a labile supercomplex in Barth syndrome patients’ cells, causing complex IV to dissociate readily from the supercomplex [17] . In various types of heart failure, excessive sympathetic stimulation may also dysregulate mitochondrial function by affecting either individual complexes or their supramolecular assemblies [18] . Recently, respiratory supercomplex factor 1 (Rcf1) and its homologue Rcf2 have been identified in yeast as factors required for the normal assembly and complete enzymatic activity of complex IV [19] , [20] , [21] . Rcf1 and Rcf2 are both required for complete complex IV assembly and enzyme activity. Rcf1 is required for complex assembly of subunits Cox13 (mammalian Cox6a) and Rcf2, as well as for the oligomerization of a subclass of cytochrome oxidase complexes into respirasomes. COX6a has been shown to be involved in the stabilization of the dimeric state of COX at a later stage of complex IV assembly, together with COX7a or COX7b subunits, and may contribute to the formation of an interaction site for cytochrome c (ref. 4 ). In the absence of Rcf1 and Rcf2, the assembly of Cox13 and Cox12 (mammalian Cox6b) are adversely affected, but the core of complex IV can associate with complex III (ref. 19 ). Thus, the Rcf1 and Rcf2 proteins are rather assumed to be complex IV late-stage assembly factors. Yet, factors responsible for supercomplex assembly per se have not been well characterized. Here we focus our study on a COX-related molecule, cytochrome c oxidase (COX) subunit 7a-related protein (COX7RP), which was originally identified as an oestrogen-responsive gene in MCF7 cells [22] . COX7RP encodes a 114-amino-acid protein, which is similar to the mitochondrial respiratory enzyme COX subunit 7a (ref. 23 ). In the present study, we assess whether COX7RP is a novel modulator of mitochondrial metabolism in vivo . We generate Cox7rp -knockout mice ( Cox7rp KO) and show that homozygous KO mice have muscle weakness. Biochemically, these animals exhibit decreased mitochondrial respiratory activities and impaired formation of mitochondrial supercomplexes in muscles. Cox7rp KO mice also exhibit heat production failure in the cold. In contrast, COX7RP -transgenic mice ( COX7RP -Tg) exhibit increased exercise performance with increased COX activity. Thus, COX7RP is shown to be a factor that functions in supercomplex assembly, which is necessary for the full activity of mitochondrial respiration. COX7RP promotes oxidative phosphorylation and ATP synthesis COX7a-related protein (COX7RP) is an oestrogen-responsive gene identified by genomic-binding site cloning [22] . Compared with the COX7a in complex IV, the amino-acid residues of the COX7RP protein are highly conserved [23] , suggesting its role in mitochondrial oxidative phosphorylation. We generated Cox7rp KO mice from the library of embryonic stem cells harbouring mutations by random retroviral gene trapping [24] . Genomic sequencing showed that the retroviral vector (7.4 kb) was inserted into the first intron of mouse Cox7rp , ( Fig. 1a ). The resulting integration caused the disruption of full-length transcripts of Cox7rp gene and the production of 2 fusion transcripts, a 5′ portion with neo and a 3′ portion with BTK. Cox7rp protein was abolished in Cox7rp KO mouse embryonic fibroblasts (MEFs) ( Fig. 1c ). In general, Cox7rp KO mice were obtained with the expected Mendelian frequency and without sexual bias. Both male and female Cox7rp KO mice were fertile and their appearance was not overtly different from that of wild-type (WT) littermates; however, COX activity and mitochondrial ATP production rate were reduced in Cox7rp KO MEFs compared with WT MEFs ( Fig. 1d ). Adenovirus-mediated introduction of COX7RP elevated COX activity and ATP production. DNA amounts in WT MEF cultures increased steadily over time, whereas those in Cox7rp KO MEFs only slightly increased over time ( Fig. 1f ). Furthermore, cellular ATP production was substantially reduced in Cox7rp KO MEFs compared with controls ( Fig. 1g ). Oxygen consumption rates dependent on complex I (pyruvate and malate as substrates), complex II (succinate as a substrate) and complex IV ( N , N , N ′, N ′-tetramethyl- p -phenylenediamine dihydrochloride, ascorbate, and carbonyl cyanide- p -trifluoromethoxyphenylhydrazone as substrates) were significantly impaired in Cox7rp KO MEFs compared with controls ( Fig. 1h ). We also generated transgenic mice that overexpress human COX7RP under the control of CAG promoter ( COX7RP -Tg, Supplementary Fig. S1a,b ). COX7RP -Tg mice were also obtained with the expected Mendelian frequency and without sexual bias. Both male and female COX7RP -Tg mice were fertile and their appearance was not overtly different from that of WT littermates. COX7RP -Tg: Cox7rp KO (TgKO) mice were generated by intercross mating between COX7RP -Tg and Cox7rp KO mice. Both male and female COX7RP -Tg mice were also apparently normal. COX7RP mRNA was increased in skeletal muscle and brown adipose tissue (BAT) of COX7RP -Tg mice ( Supplementary Fig. S1c,d ). COX activity and cell proliferation ability were enhanced in COX7RP -Tg MEFs compared with WT MEFs ( Supplementary Fig. S1e,f ). 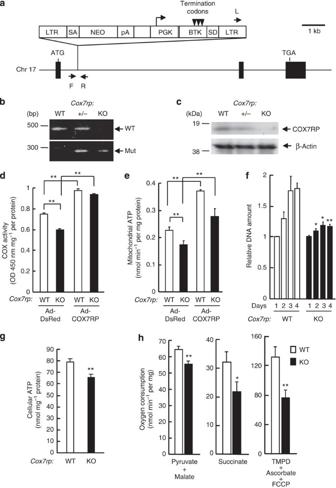Figure 1:Reduction of mitochondrial respiratory activity in MEFs derived fromCox7rpKO mice. (a) Generation ofCox7rpKO mice. Schematic representation of the gene trap vector insertion site in the mutant gene. BTK, bruton tyrosine kinase cassette; LTR, long terminal repeat; NEO, neomycin-resistant gene cassette; pA, polyadenylation sequence; PGK, phosphoglycerate kinase-1 promoter; SA, splicing acceptor site; SD, splicing donor site. (b) Genotyping ofCox7rpKO mice. Representative litters containing WT,Cox7rp+/−(+/−) andCox7rpKO (KO) mice were shown. Sense primer-F and -L within intron 1 and the vector, and common antisense primer-R within intron 1 (a) were used to amplify WT (489 bp) and mutant (Mut: 289 bp) alleles, respectively. (c) Western blot analysis ofCox7rpKO MEFs. Cell extracts from MEFs were resolved on SDS–polyacrylamide gel and immunoblotted with anti-COX7RP. (d) Decrease in COX activity inCox7rpKO MEFs. COX activity was assessed using MEFs from WT andCox7rpKO mice infected with recombinant adenovirus expressing control DsRed (Ad-DsRed) or COX7RP (Ad-COX7RP). Data are presented as means±s.d. (n=3). *P<0.05 for WT versus KO; Student’st-test. (e) Decrease in mitochondrial ATP production inCox7rpKO MEFs. ATP production was assessed using MEFs from WT andCox7rpKO mice infected with Ad-DsRed or Ad-COX7RP. Data are presented as means±s.d. (n=3). *P<0.05 for WT versus KO; Student’st-test. (f) Retardation of growth inCox7rpKO MEFs. Data are presented as means±s.d. (n=3). *P<0.05, **P<0.01 for WT versus KO at each indicated time point; Student’st-test. (g) Decline of cellular ATP content inCox7rpKO MEFs. Data are presented as means±s.d. (n=3). **P<0.01 for WT versus KO; Student’st-test. (h) Decreased oxygen consumption rates ofCox7rpKO MEFs. MEFs were permeabilized with digitonin, and subsequently substrates and inhibitors were added. Rates of oxygen consumption are expressed as nanomoles of oxygen per minute per milligram of protein. Data are presented as means±s.d. (n=3) *P<0.05, **P<0.01 for WT versus KO under each condition; Student’st-test. Figure 1: Reduction of mitochondrial respiratory activity in MEFs derived from Cox7rp KO mice. ( a ) Generation of Cox7rp KO mice. Schematic representation of the gene trap vector insertion site in the mutant gene. BTK, bruton tyrosine kinase cassette; LTR, long terminal repeat; NEO, neomycin-resistant gene cassette; pA, polyadenylation sequence; PGK, phosphoglycerate kinase-1 promoter; SA, splicing acceptor site; SD, splicing donor site. ( b ) Genotyping of Cox7rp KO mice. Representative litters containing WT, Cox7rp +/− (+/−) and Cox7rp KO (KO) mice were shown. Sense primer-F and -L within intron 1 and the vector, and common antisense primer-R within intron 1 ( a ) were used to amplify WT (489 bp) and mutant (Mut: 289 bp) alleles, respectively. ( c ) Western blot analysis of Cox7rp KO MEFs. Cell extracts from MEFs were resolved on SDS–polyacrylamide gel and immunoblotted with anti-COX7RP. ( d ) Decrease in COX activity in Cox7rp KO MEFs. COX activity was assessed using MEFs from WT and Cox7rp KO mice infected with recombinant adenovirus expressing control DsRed (Ad-DsRed) or COX7RP (Ad-COX7RP). Data are presented as means±s.d. ( n =3). * P <0.05 for WT versus KO; Student’s t -test. ( e ) Decrease in mitochondrial ATP production in Cox7rp KO MEFs. ATP production was assessed using MEFs from WT and Cox7rp KO mice infected with Ad-DsRed or Ad-COX7RP. Data are presented as means±s.d. ( n =3). * P <0.05 for WT versus KO; Student’s t -test. ( f ) Retardation of growth in Cox7rp KO MEFs. Data are presented as means±s.d. ( n =3). * P <0.05, ** P <0.01 for WT versus KO at each indicated time point; Student’s t -test. ( g ) Decline of cellular ATP content in Cox7rp KO MEFs. Data are presented as means±s.d. ( n =3). ** P <0.01 for WT versus KO; Student’s t -test. ( h ) Decreased oxygen consumption rates of Cox7rp KO MEFs. MEFs were permeabilized with digitonin, and subsequently substrates and inhibitors were added. Rates of oxygen consumption are expressed as nanomoles of oxygen per minute per milligram of protein. Data are presented as means±s.d. ( n =3) * P <0.05, ** P <0.01 for WT versus KO under each condition; Student’s t -test. Full size image Cox7rp null mice have reduced running endurance In 4-month-old Cox7rp KO mice, the weights of quadriceps femoris muscles were reduced compared with WT littermates, although the body weights were not significantly different ( Supplementary Fig. S2a,b ). Histochemical staining revealed a reduction of COX activity in quadriceps femoris muscles of 4-month-old Cox7rp KO mice, whereas COX activity was restored in a cross-bred strain of COX7RP -Tg: Cox7rp KO (TgKO) ( Fig. 2a ). COX activities in quadriceps femoris, gastrocnemius and cardiac muscles of KO mice were 15–30% reduced compared with WT littermates ( Supplementary Fig. S3 ). In the forced treadmill test, Cox7rp KO mice showed 70% of the running capacity of their age- and weight-matched WT counterparts ( Fig. 2b , Supplementary Fig. S4 and Supplementary Movies 1–4 ). COX7RP -Tg mice exhibited 130% of the running capacity of WT mice and TgKO mice recovered the running ability to the level of WT mice. Expression microarray analysis revealed the dysregulation of pathways involved in muscle physiology and diseases in Cox7rp KO muscles ( Supplementary Tables S1 and S2 ). Thus, Cox7rp loss-of-function leads to reduced mitochondrial oxidative capacity and impaired muscle function in response to forced physical exertion. In the study of indirect calorimetry during treadmill exercise, Cox7rp KO had lower CO 2 production (VCO 2 ) and O 2 consumption (VO 2 ), while the respiration quotient (RQ) was higher compared with WT controls ( Fig. 2c ), indicating a decrease in the metabolic rate and a metabolic shift to glucose consumption. Reduction of VO 2 and VCO 2 in Cox7rp KO mice was also shown in the steady state before exercise ( Supplementary Fig. S5 ). In contrast, COX7RP -Tg mice exhibited an increase in VO 2 and VCO 2 even in the steady state. 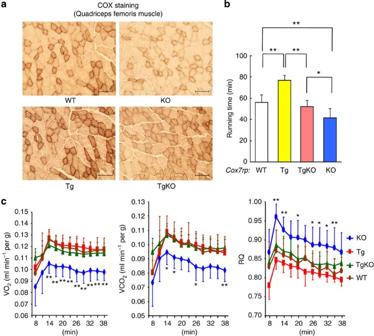Figure 2:Reduction of COX activity in muscles and compromised exercise performance inCox7rpKO mice. (a) Reduced COX activity inCox7rpKO mice. COX staining of the quadriceps femoris of 4-month-old WT,Cox7rpKO (KO),COX7RP-Tg (Tg) andCOX7RP-Tg:Cox7rpKO (TgKO) mice. Scale bar, 100 μm. (b) Compromised exercise performance inCox7rpKO mice. Four-month-old KO, Tg and TgKO mice, as well as WT controls were subjected to a forced treadmill exercise test. Data are presented as means±s.d. (n=7 or 8). *P<0.05, **P<0.01; Dunnett’spost hoctest. (c) Increase in the respiration quotient inCox7rpKO mice. CO2production, O2consumption and RQ were analysed during the above treadmill exercise test. Data are presented as means±s.d. (n=7 or 8). *P<0.05, **P<0.01; Dunnett’spost hoctest. Figure 2: Reduction of COX activity in muscles and compromised exercise performance in Cox7rp KO mice. ( a ) Reduced COX activity in Cox7rp KO mice. COX staining of the quadriceps femoris of 4-month-old WT, Cox7rp KO (KO), COX7RP -Tg (Tg) and COX7RP -Tg: Cox7rp KO (TgKO) mice. Scale bar, 100 μm. ( b ) Compromised exercise performance in Cox7rp KO mice. Four-month-old KO, Tg and TgKO mice, as well as WT controls were subjected to a forced treadmill exercise test. Data are presented as means±s.d. ( n =7 or 8). * P <0.05, ** P <0.01; Dunnett’s post hoc test. ( c ) Increase in the respiration quotient in Cox7rp KO mice. CO 2 production, O 2 consumption and RQ were analysed during the above treadmill exercise test. Data are presented as means±s.d. ( n =7 or 8). * P <0.05, ** P <0.01; Dunnett’s post hoc test. Full size image COX7RP regulates heat production in BAT BAT weights of WT and COX7RP -Tg mice were almost the same, whereas Cox7rp KO BAT was substantially enlarged with white adipose tissue-like appearance, resulting from the accumulation of lipid droplets ( Fig. 3a , and Supplementary Fig. S2c ). The weights of BAT in TgKO mice were intermediate. In the temperature challenge study, Cox7rp KO mice showed severe cold sensitivity 4 h after cold exposure at 4 °C, whereas WT mice could maintain their body temperature under the same condition ( Fig. 3c ). In the cold exposure study in which the experimental end point was the body temperature ≤15 °C, Cox7rp KO mice exhibited the shortest dropout time among the four genotypes ( Fig. 3d ). Notably, the mRNA level of uncoupling protein Ucp1 , which is known to have a critical role in the energy dissipation in BAT, was severely decreased in Cox7rp KO BAT ( Fig. 3e ). Expression microarray analysis revealed the dysregulation of pathways involved in mitochondria metabolism, oxidation and reduction reactions, fatty acid and lipid metabolism, and fat cell differentiation in Cox7rp KO BAT ( Supplementary Tables S3 and S4 ). Thus, disruption of Cox7rp function leads to transition of BAT to white adipose tissue-like structure and thermogenic defects in cold environments. In addition, by assessing expression levels of transcriptional regulatory factors crucial for mitochondrial function, Pparα, Pparγ, Pgc-1α and Pgc-1β were revealed to be downregulated in BAT of Cox7rp KO mice ( Supplementary Fig. S6 ). 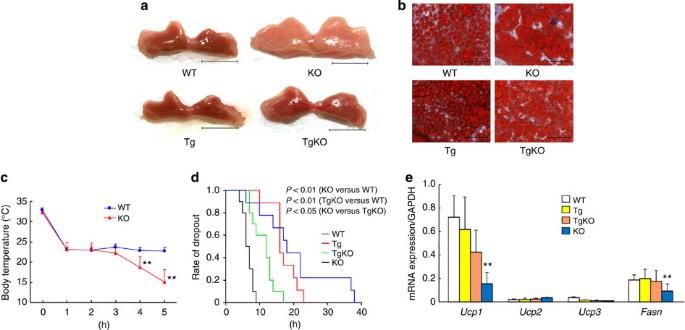Figure 3:Increased mass and fat droplets of BAT and impaired resistance to cold exposure inCox7rpKO mice. (a) Appearance of brown fat pads of 4-month-old WT, KO, Tg and TgKO mice. Scale bar, 5 mm. (b) Histological section and oil red O staining of brown fats of 4-month-old WT, KO, Tg and TgKO mice. Scale bar, 100 μm. (c)Cox7rpKO mice are cold-sensitive. Body temperature of WT (blue box) andCox7rpKO (red triangle) mice exposed to 4 °C for 5 h was measured by using a thermofocus infrared thermometer. Data are the means±s.d. of five animals per group. **P<0.01; Student’st-test. (d) COX7RP-Tg mice demonstrate improved cold tolerance. Kaplan–Meier analysis of the body temperature was performed for mice exposed to 4 °C for 5 h, in which the end point was defined as ≤15 °C (n=7 or 8). Log-rankP-values after application of a Bonferroni correction were indicated. (e) Decreased mRNA expression of uncoupling proteins and fatty acid synthase (Fasn) inCox7rpKO BAT. qPCR analysis was performed using total RNA from WT, KO, Tg and TgKO BAT. **P<0.01; Dunnett’spost hoctest. Figure 3: Increased mass and fat droplets of BAT and impaired resistance to cold exposure in Cox7rp KO mice. ( a ) Appearance of brown fat pads of 4-month-old WT, KO, Tg and TgKO mice. Scale bar, 5 mm. ( b ) Histological section and oil red O staining of brown fats of 4-month-old WT, KO, Tg and TgKO mice. Scale bar, 100 μm. ( c ) Cox7rp KO mice are cold-sensitive. Body temperature of WT (blue box) and Cox7rp KO (red triangle) mice exposed to 4 °C for 5 h was measured by using a thermofocus infrared thermometer. Data are the means±s.d. of five animals per group. ** P <0.01; Student’s t -test. ( d ) COX7RP-Tg mice demonstrate improved cold tolerance. Kaplan–Meier analysis of the body temperature was performed for mice exposed to 4 °C for 5 h, in which the end point was defined as ≤15 °C ( n =7 or 8). Log-rank P- values after application of a Bonferroni correction were indicated. ( e ) Decreased mRNA expression of uncoupling proteins and fatty acid synthase (Fasn) in Cox7rp KO BAT. qPCR analysis was performed using total RNA from WT, KO, Tg and TgKO BAT. ** P <0.01; Dunnett’s post hoc test. Full size image COX7RP is involved in respiratory supercomplex assembly We next investigated the contribution of COX7RP to supercomplex assembly. In two-dimensional blue native polyacrylamide gel electrophoresis (PAGE) with subsequent immunoblotting for digitonin-solubilized mitochondria in muscles, Cox7rp was detected predominantly in I/III 2 /IV n supercomplex in WT but not in Cox7rp KO mitochondria ( Fig. 4a ). Intensity of Cox4 signal in supercomplex I/III 2 /IV n was significantly reduced by Cox7rp loss, as ~50 and 5% of Cox4 were involved in the supercomplex of WT and KO mitochondria, respectively. We also noted that Cox4 signal in monomeric complex IV was increased, whereas the signal in dimeric complex IV was decreased in Cox7rp KO mitochondria. In terms of complex III assembly, the signal of Rieske iron-sulfur protein (Risp), a late-stage subunit of supercomplex [25] , was decreased in I/III 2 /IV n in Cox7rp KO muscle compared with WT muscle ( Fig. 4c ). An overexpression study of COX7RP in 293T cells also revealed that COX7RP has a role in stabilizing complex IV dimerization and supercomplex assembly (Supplementary Fig. S7a,b). The RISP signal in I/III 2 /IV n supercomplex was substantially intense in COX7RP-overexpressing cells compared with control cells ( Supplementary Fig. S7c,d ). Taken together, the data reveal that COX7RP is a promoting factor for the organization of I/III 2 /IV n supercomplex. The contribution of COX7RP to the assembly of III 2 /IV n supercomplex is not clear so far based on our results. 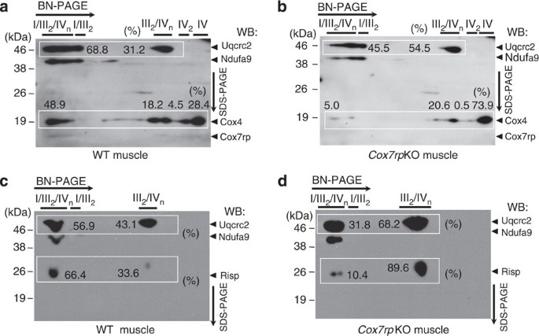Figure 4: COX7RP promotes assembly of respiratory chain supercomplexes. Mitochondrial proteins of skeletal muscle from WT (a,c) andCox7rpKO mice (b,d) were solubilized with digitonin in the concentration of 2 g g−1protein (a,b) or 0.5 g g−1protein (c,d), and subjected to blue native polyacrylamide gel electrophoresis (BN-PAGE) followed by second-dimensional SDS–PAGE. Western blot analysis was performed with antibodies for NDUFA9 of complex I, UQCRC2 of complex III, RISP of complex III, COX4 of complex IV and COX7RP. Positions corresponding to mitochondrial supercomplex species I/III2/IVn, I/III2, III2/IVn, dimerized complex IV (IV2) and monomerized complex IV (IV) are indicated. Percentages of UQCRC2, RISP or COX4 signal intensities in each whole amount are indicated in the images. Figure 4: COX7RP promotes assembly of respiratory chain supercomplexes. Mitochondrial proteins of skeletal muscle from WT ( a , c ) and Cox7rp KO mice ( b , d ) were solubilized with digitonin in the concentration of 2 g g −1 protein ( a , b ) or 0.5 g g −1 protein ( c , d ), and subjected to blue native polyacrylamide gel electrophoresis (BN-PAGE) followed by second-dimensional SDS–PAGE. Western blot analysis was performed with antibodies for NDUFA9 of complex I, UQCRC2 of complex III, RISP of complex III, COX4 of complex IV and COX7RP. Positions corresponding to mitochondrial supercomplex species I/III 2 /IV n , I/III 2 , III 2 /IV n , dimerized complex IV (IV 2 ) and monomerized complex IV (IV) are indicated. Percentages of UQCRC2, RISP or COX4 signal intensities in each whole amount are indicated in the images. Full size image Our findings provide a new insight into the normal and pathological relevance of mitochondrial supercomplex assembly in mammalian systems. COX7RP is a nuclear DNA-encoded mitochondrial gene that can facilitate supercomplex assembly of the mitochondrial respiratory chain and can modulate mitochondrial energy metabolism. The characteristics of Cox7rp KO mice reveal that the gene has a critical role in muscle activity, as well as adaptive thermogenesis in vivo . The present study demonstrates the first mammalian phenotype of the disorder of a supercomplex-promoting factor, which enables researchers to dissect the function of COX7RP in normal and disease states of mitochondria and to manipulate the structure of supercomplex assembly in vivo . As structurally COX7RP-related proteins, COX7A family originally contains two members, COX7A1 and COX7A2 (ref. 26 ). COX7A has been shown as one of the 13 subunits of bovine heart complex IV by crystal structure analysis [4] . KO mice of heart-type Cox7a1 showed reduced COX activity, dilated cardiomyopathy at 6 weeks of age [27] and resulted in exercise intolerance [28] . These findings indicate that COX7A family may have important roles in COX activity and its regulation; however, the precise molecular mechanism has not been understood. COX7A has been considered as a late-assembling subunit similar to COX6A ref. 29 , and in vitro translated COX7A was first incorporated into complex IV and supercomplex III+IV based on in vitro import and assembly assays [30] . Thus, it is likely that COX7A has a role in the late steps of holo-complex IV formation, as well as in the assembly of III and IV, and is located in the periphery of complex IV. In regard to the stoichiometry of COX7A in complex IV, either COX7A1 or COX7A2 would be involved in complex IV as preferential expression of COX7A1 and COX7A2 are known in muscles and liver, respectively. Compared with other COX7A family proteins, COX7RP protein harbours a specific N-terminal domain through which COX7RP may exert unique function in the regulation of supercomplex assembly and mitochondrial respiration. Our data reveal that COX7RP is a unique factor that promotes the assembly of supercomplex III+IV with complex I, (as opposed to the assembly of III and IV). Considering possible differential functions of COX7RP and COX7A, COX7RP might exist in the more peripheral region of complex IV after the incorporation of COX7A into complex IV, and both COX7RP and a tissue-specific COX7A may be incorporated into complex IV or supercomplex I/III/IV. It is also speculated that once COX7RP binds to supercomplex III+IV, it would be quickly incorporatred into supercomplex I/III/IV as COX7RP may function as a pilot. It may be one reason why the role of COX7RP in the assembly of III and IV has not been clearly shown in our results. Questions are still remained whether COX7A also has a role in the assembly of supercomplex III+IV with I and whether COX7A can substitute for COX7RP in this context. Taken together, COX7A and COX7RP may have distinct roles in supercomplex assembly, as COX7A supports COX assembly in the III 2 /IV n supercomplex, while COX7RP supports COX's ability to assemble with III into the I/III 2 /IV n supercomplex. We found that the brown adipocytes in Cox7rp KO mice accumulate excess amounts of lipids, resulting in a cold-sensitive phenotype of KO mice. BAT is an essential tissue that contains abundant mitochondria and exerts energy dissipation and rapid thermogenesis through mitochondrial uncoupling, utilizing uncoupling proteins such as UCP1 (refs 31 , 32 ). Ucp1 and Fasn mRNA expression is impaired in Cox7rp KO BAT. Thus, COX7RP has a critical role in heat production or lipid metabolism in BAT. It is also notable that RQ in Cox7rp KO mice is elevated during exercise. The result implies that COX7RP may be preferentially involved in the utilization of fatty acids or amino acids rather than glucose in a condition demanding high production of energy. Future study of Cox7rp KO and COX7RP -Tg mice fed with high- or low-fat diet will further provide information in regard to the contribution of COX7RP to glucose and lipid metabolism, obesity, insulin resistance and diabetes. Interestingly, a couple of mice models deficient in genes related to energy metabolism also exhibit impaired thermogenesis, similar to Cox7rp KO mice. Mice lacking oestrogen-related receptor alpha (ERRα) are defective in adaptive thermogenesis due to the reduction of mitochondrial mass and oxidative capacity in brown adipocytes [33] , as this nuclear receptor is considered as an important transcription factor that regulates mitochondrial biogenesis and oxidative metabolism [34] , [35] . The ERRα coactivator peroxisome proliferator-activated receptor-gamma coactivator 1α (PGC-1α) has been also shown to regulate adaptive thermogenesis in BAT [36] , [37] , [38] . Increased expression of PGC-1α delays the onset of mitochondrial myopathy in mice with skeletal muscle-targeted ablation of the COX assembly factor COX10 (ref. 39 ). Increased expression of PGC-1β, as well as PGC-1α improved mitochondrial respiration in cells with complex III or IV deficiency [40] . These studies may indicate that COX7RP is one of the genes involved in pathways regulated by ERRα and PGC-1α. Indeed, Cox7rp has been shown to be one of the downregulated metabolic genes in a heart failure mouse model with cardiac-specific disruption of Cdk7/cyclin H/ménage-à-trois 1, which is critical for the transcriptional function of PGC-1α (ref. 41 ). Impaired mitochondrial activity due to Cox7rp loss may also lead to the altered expression of nuclear-encoded mitochondrial genes, as we found that Pgc-1α and β mRNA expressions were downregulated in Cox7rp KO BAT. It has been known that mitochondrial dysfunction can activate retrograde signalling from mitochondria to the nucleus, which has a role in life span expansion in yeasts, for example [42] . In mitochondrial dysfunction, cellular NAD+/NADH ratio, ATP/ADP ratio, cytosolic free Ca 2+ concentration, cellular oxidative stress may act as signalling mediators that modulate the downstream transcription factors in the nucleus [43] . In particular, PGC-1α has important roles in mitochondrial retrograde signalling. For example, the transcription of PGC-1α gene is activated by phosphorylated CREB transcription coactivator triggered by increased cytosolic Ca 2+ (ref. 44 ). Cellular stress-dependent ATP depletion activates AMP-activated protein kinase, which also phosphorylates and activates PGC-1α (ref. 45 ). In mammalian cells with an A3242G mutation of mitochondrial DNA, mitochondrial dysfuction altered expressions of several transcription factors including RXRA, which led to the decrease in PGC-1α recruitment and the repression of oxidative phosphorylation genes [46] . The involvement of PGC-1β in the retrograde signalling has not been reported, however, Pgc-1β may also have a role in the pathological condition of Cox7rp KO mice similar to Pgc-1α. In conclusion, COX7RP is a nuclear DNA-encoded mitochondrial gene that can promote the respiratory supercomplex assembly of the III 2 /IV n supercomplex with complex I, rather than the assembly of the III 2 /IV n supercomplex itself. COX7RP has a critical role in muscle activity, as well as adaptive thermogenesis in vivo . Our different mouse strains with altered COX7RP expression will be useful tools for modulating the state of supercomplex assembly and exploring energy metabolism in normal and disease states. Anti-COX7RP polyclonal antibody A polyclonal antibody against COX7RP was raised in rabbits as described previously [47] . Briefly, a peptide that comprised 14 amino-acid residues corresponding with the C-terminal region of human COX7RP protein was used to immunize Japanese white rabbits. The serum was affinity purified using Affigel 10 (Bio-Rad) according to the manufacturer’s instructions. COX activity The COX activity in cultured cells was assessed as described elsewhere [48] . Briefly, cells permeabilized with 0.01% saponin were incubated for 15 min in 4 nM 3,3′-diaminobenzidine tetra hydrocholoride (DAB) (Sigma), 100 μM reduced cytochrome c (Sigma), 2 μg ml −1 of catalase (Sigma) in 0.1 M phosphate buffer, pH 7.0. Absorbance was measured using a 450-nM filter. Muscle homogenates were also applied to the COX activity-measuring method described above. For the histological study of COX activity, cross-sections (10 μm thick) of frozen muscles were stained as described above. ATP synthesis ATP synthesis in mitochondria was measured as described previously [49] . Briefly, cells were incubated in 150 mM KCl, 25 mM Tris-HCl, pH 7.4, 2 mM EDTA, 10 mM potassium phosphate, 0.1 mM MgCl 2 and 0.1% bovine serum albumin, supplemented with 50 μg ml −1 digitonin. Mitochondria were energized using 1 mM malate and 1 mM pyruvate as substrates in the presence of 1 mM ADP and 0.15 mM adenylate kinase inhibitor P1,P5- di(adenosine-5′)pentaphosphate and incubated for 10 min at 37 °C. Parallel incubations were also carried out in the presence of 2 μg ml −1 oligomycin to measure mitochondria-specific ATP synthesis. ATP was measured by using the Enliten assay system (Promega). Mice and MEF preparation Cox7rp KO mice were generated by Lexicon Genetics using random retroviral gene trapping in ES cells as previously described [24] . Cox7rp KO mice were born at Mendelian ratios and were fertile. Two pairs of Cox7rp heterozygous mice were purchased and backcrossed to the C57BL/6 inbred strain through nine generations to generate Cox7rp -deficient mice and WT littermates used. The genotype of Cox7rp KO mice was determined by using PCR. Three primers, named F, R and L, were designed based on the genomic sequence surrounding the insertion site and the sequence of vector-specific oligonucleotides. Primer sequences were as follows: Primer-F, 5′-TCTGGTTGAGGTGGCCTTTGTGACTT-3′; Primer-R, 5′-TTATCCAGCACCAACCATCTGCCAGA-3′; and Primer L, 5′-AAATGGCGTTACTTAAGCTAGCTTGC-3′. CAG- Flag -tagged COX7RP transgene plasmid was constructed using pCXN2 vector that contains CAG promoter, being a composite promoter consisting of a cytomegalovirus IE enhancer, a chicken β-actin promoter, two functional loxP sites and a rabbit β-globin polyadenylation signal [50] . CAG- Flag -tagged COX7RP plasmid was linearized by restriction enzyme digestion. Transgenic mice were produced by microinjection of the linearized plasmid into the pronuclei of fertilized eggs from C57BL/6 mice as described previously [51] . Transgenic mice were identified by PCR of genomic DNA extracted from the tail. Primers derived from the 5′- and 3′-flanking sequences of CAG promoter and polyA signal (5′-CCTACAGCTCCTGGGCAACGTGCTGGTT-3′ and 5′-AGAGGGAAAAAGATCTCAGTGGYAY-3′) were used to amplify a 600-bp product. Cox7rp -TgKO mice were generated by intercross mating between Cox7rp KO and COX7RP -Tg mice. MEFs were obtained from 16-day-old embryos of WT, Cox7rp KO and COX7RP -Tg mice and used at two to three generations. For assays of COX activity and mitochondrial ATP synthesis, MEFs were infected with a recombinant adenovirus expressing COX7RP (Ad-COX7RP) or the fluorescent protein DsRed (Ad-DsRed) at a multiplicity of infection of 10 for 48 h. The adenoviral vectors were constructed using the Adenovirus Expression Vector Kit (Takara, Tokyo, Japan) following the manufacturer’s protocol. All mice used for the experiments were maintained in a specific pathogen-free mouse facility. All studies involving animals were reviewed and approved by the Institutional Animal Care and Use Committee of Siatama Medical University. Indirect calorimetry analysis in exercised and rested conditions The respiratory metabolic rate was measured using an individual open-circuit indirect calorimetric system equipped with an airtight treadmill (TREADMILL FOR MICE MODEL MK-680AT/O 2 M, Muromachi, Japan). Before the exercise performance test, mice were accustomed to the treadmill by subjecting them to a 3-min run at 10 m min −1 once per day for 2 days. The exercise test regimen was 15 m min −1 for the first 10 min, followed by an incremental increase of 2 m min −1 at 10-min intervals. Exhaustion was defined as a state when the mice were unable to avoid repetitive electrical shocks. The respiratory metabolic rate was also measured in the non-exercise condition using an indirect calorimetric system equipped with an airtight metabolic chamber (Muromachi, Japan) for 1 h. During this time, the data for each chamber were collected every 3 min with room air as reference to calculate CO 2 production, O 2 consumption and RQ. Oxygen consumption rate measurements Oxygen consumption rates were measured using a Strathkelvin 1302 oxygen electrode with an MT200 Mitocell respiration chamber (Strathkelvin Instruments Ltd, Glasgow, UK) at 37 °C. Trypsinized cells were resuspended in KCl medium containing 80 mM KCl, 10 mM Tris-HCl (pH 7.4), 3 mM MgCl 2 , 1 mM EDTA and 5 mM potassium phosphate and permeabilized with digitonin (0.05 mg mg −1 protein). Substrates and inhibitors were added in the following order and final concentration: 10 mM pyruvate+2 mM malate+2 mM ADP as complex I substrates, 5 μM rotenone as complex I inhibitor, 10 mM succinate as complex II substrate, 4 μM antimycin A as complex III inhibitor and 2 mM ascorbate+0.5 mM N , N , N ′, N ′-tetramethyl- p -phenylenediamine dihydrochloride+0.5 μM carbonyl cyanide- p -trifluoromethoxyphenylhydrazone as complex IV substrates in uncoupled respiration. Rates of oxygen consumption are expressed as nanomoles of oxygen per minute per milligrams of protein. Oil red O staining Interscapular BAT was fixed in 4% PBS-buffered paraformaldehyde solution and frozen in liquid nitrogen. Thirty-micrometer-thick sections were stained with oil red O and counter-stained with hematoxylin. Thermogenic response to cold exposure For acute cold exposure experiments, 4-month-old WT, Cox7rp KO and COX7RP -Tg littermates were transferred to 4 °C and body temperature was measured every 60 min at the tail base using a thermofocus infrared thermometer (Tecnimed, Varese, Italy) until any of the mice showed hypothermia (tail base temperature ≤15 °C). Blue native PAGE Skeletal muscle or 293T cells transfected with COX7RP or vector were homogenized with a glass-teflon homogenizer in buffer containing 10 mM HEPES-KOH (pH 7.4), 0.22 M mannitol, 0.07 M sucrose and 0.1 mM EDTA. Cell extracts were centrifuged at 500 g and the mitochondrial fraction was precipitated by further centrifugation at 8,000 g . Mitochondria (100 μg mitochondria protein) were suspended in 10 μl of a buffer containing 50 mM Bis-Tris and 1 M 6-aminocaproic acid. Digitonin (digitonin/protein ratio of 0.5–2 g g −1 ) was added to solubilize the mitochondria. As RISP is known as a late-stage assembly subunit in mitochondrial respiratory supercomplex [25] , a milder solubilization condition of 0.5 g digitonin per gram protein was employed to detect RISP. After 30-min incubation at 4 °C, the solubilized proteins were obtained as supernatant fraction by centrifugation at 22,000 g . The solubilized proteins were supplemented with 1 μl of sample buffer (5% Coomassie brilliant blue G-250 in 0.5 M 6-aminocaproic acid). A stacking gel (4%) and separating gels with a stepwise 8, 9, 10 and 11% were cast and electrophoresed according to the method of Schägger and von Jagow [52] . The second-dimension SDS–PAGE and immunoblotting were performed according to standard protocols, and the blot was probed with anti-NDUFA9 (Invitrogen) and anti-UQCRC2 antibodies (Abcam), together with anti-COX7RP anti-COX4 antibodies (Cell Signaling) or with anti-RISP antibody (Abcam). Experiments were carried out four times and representative results are shown in figures. full-length images of immunoblots are shown in Supplementary Fig. S8 . Quantitative real-time polymerase chain reaction Total RNA was extracted from the BAT of 4-month-old WT and Cox7rp KO male mice using the ISOGEN reagent (Nippon Gene, Tokyo, Japan). Quantitative real-time RT–PCR (qPCR) analysis was performed as described previously [53] . The sequences of the PCR primers used were as follows: common primers for human and mouse Cox7rp , 5′-GTTCCACAGAAGCACCACCTATC-3′ and 5′-GGTCCGGTAAAGCATTTGGTC-3′; mouse specific Cox7rp , 5′-GCAGAAGTTGGCTGGAGCTT-3′ and 5′-TATGCTGTCACACTGGAGGTCAG-3′; Ucp1 , 5′-CGTACCAAGCTGTGCGATGT-3′ and 5′-ACCCGAGTCGCAGAAAAGAA-3′; Ucp2 , 5′-AACTCTGCCTTGGGCCAGTAC-3′ and 5′-CGGAGAAAGGAAGGCATGAA-3′; Ucp3 , 5′-TTGGCCTCTACGACTCTGTCAA-3′ and 5′-ATGGCTTGAAATCGGACCTTC-3′; Fasn , 5′-GCTGTCCCCTGATGCCATT-3′ and 5′-ACCTATCCCGGCCTGAGAAC-3′; Pparα , 5′-GATCGGCCTGGCCTTCTAA-3′ and 5′-GGTGTCATCTGGATGGTTGCT-3′; Pparγ , 5′-TTCCGAAGAACCATCCGATT-3′ and 5′-TTTGTGGATCCGGCAGTTAAG-3′; Pparδ , 5′-ACACCATTCTGCGGGCTCTA-3′ and 5′-GGGAAGAGGTACTGGCTGTCAG-3′; Pgc-1α , 5′-GGCACGCAGCCCTATTCAT-3′ and 5′-CACGGAGAGTTAAAGGAAGAGCAA-3′; Pgc-1β , 5′-CATCTGGGAAAAGCAAGTACGA-3′ and 5′-CCTCGAAGGTTAAGGCTGATATCA-3′; Errα , 5′-GGAGTACGTCCTGCTGAAAGCT-3′ and 5′-CACAGCCTCAGCATCTTCAATG-3'; Errβ , 5′-CGATATCCCCGAGGGAGATATC-3′ and 5′-CCAGTTGATGAGGAACACAAGCT-3′; Errγ , 5′-GACCCTACTGTCCCCGACAGT-3′ and 5′-AACTCTCGGTCAGCCAAGTCA-3′; Nrf1 , 5′-CTTACAAGGTGGGGGACAGA-3′ and 5′-CCGATATCCTGGTGGTCACT-3′; Tfam , 5′-TGGAAAGCATACAAAGAAGCTG-3′ and 5′-GACAGATTTTTCCAAGCCTCA-3′; and Gapdh , 5′-GCATGGCCTTCCGTGTTC-3′ and 5′-TGTCATCATACTTGGCAGGTTTCT-3′. Comparison of the amounts of PCR product was carried out by employing the comparative cycle threshold (Ct) method, using Gapdh as control. The experiments were independently performed in triplicate. Results were shown as means±s.d. Microarray analysis Gene expression in the muscle and BAT of 5-month-old WT and Cox7rp KO male mice was measured with Affymetrix GeneChip (Mouse Gene 1.0 ST Array) according to the manufacturer’s protocol. The DAVID Functional Annotation Clustering Tool ( http://david.abcc.ncifcrf.gov/summary.jsp ) was used to perform a global analysis of gene expression and to sort differentially expressed genes into pathways and clusters of functionally related genes. Statistics We determined the significance of differences between the two groups by using the unpaired Student’s t -test. Comparisons among several groups were carried out with one-way analysis of variance followed by Dunnett’s post hoc test. Survival analyses were carried out using Kaplan–Meier method. We considered a value of P <0.05 to be statistically significant. Bonferroni correction was used to adjust for multiple comparisons. How to cite this article: Ikeda, K. et al. A stabilizing factor for mitochondrial respiratory supercomplex assembly regulates energy metabolism in muscle. Nat. Commun. 4:2147 doi: 10.1038/ncomms3147 (2013).